Understanding the role of phase in chemical bond breaking with coincidence angular streaking Electron motion in chemical bonds occurs on an attosecond timescale. This ultrafast motion can be driven by strong laser fields. Ultrashort asymmetric laser pulses are known to direct electrons to a certain direction. But do symmetric laser pulses destroy symmetry in breaking chemical bonds? Here we answer this question in the affirmative by employing a two-particle coincidence technique to investigate the ionization and fragmentation of H 2 by a long circularly polarized multicycle femtosecond laser pulse. Angular streaking and the coincidence detection of electrons and ions are employed to recover the phase of the electric field, at the instant of ionization and in the molecular frame, revealing a phase-dependent anisotropy in the angular distribution of H + fragments. Our results show that electron localization and asymmetrical breaking of molecular bonds are ubiquitous, even in symmetric laser pulses. The technique we describe is robust and provides a powerful tool for ultrafast science. Ultrashort laser pulses are extensively employed to probe ultrafast processes, where the measurement of time intervals is usually based on the pump-probe concept. In this scheme, an ultrashort laser pulse is split into two pulses, with one being used as the pump to excite the target and the other time-delayed pulse acting as the probe. By scanning the delay between the pump and probe pulses, snapshots of the ultrafast dynamics are taken. The time measurement is realized by converting the time interval to the propagation distance of the light (~0.3 μm fs −1 in air). The femtosecond (fs) pump-probe technique is routinely applied in many fields of physics, chemistry and biochemistry [1] , [2] , [3] . The time resolution of a pump-probe experiment is generally limited by the temporal duration of the laser pulses employed. As the timescale for electronic motion is much shorter than 1 fs, attosecond (10 −18 s) pulses are required to resolve electron dynamics in a pump-probe scheme. To date however, the intensity of these pulses [4] , [5] is too low for their use in a conventional pump-probe setup. In this work, we pursue an alternative route to investigate ultrafast dynamics. Our approach is inspired by two previously used attosecond time-measurement techniques. The first technique combines a single attosecond pulse with an intense near-infrared laser pulse, such that the attosecond pulse acts as a start and the phase-locked infrared pulse streaks a freed electron in energy [6] , [7] , [8] , [9] . The second technique, termed ‘attosecond angular streaking’, uses elliptically polarized light [10] , [11] , [12] , [13] , [14] , [15] and adopts either the major axis of the elliptical field or the carrier-envelope phase (CEP) of a CEP-stabilized pulse to provide a reference time. A released electron is then driven to a certain direction by the rotating electric field, which maps the ionization instant within one laser cycle ( T p ~2.6 fs at 790 nm) to the 2 π interval of electron emission directions (~7.3 attosecond for 1°) in the polarization plane. Our technique, shown schematically in Fig. 1a , combines angular streaking with the coincident detection of two particles. Although it does not resolve time intervals on the attosecond timescale, it enables us to perform a phase- and energy-resolved study of electron localization along a molecular bond occurring through the process of molecular fragmentation. A randomly aligned ensemble of H 2 molecules is exposed to the rotating electric field of a circularly polarized long laser pulse. The first part of the pulse launches the nuclear wavepacket by releasing one electron from the neutral molecule at time t i . The second part of the same pulse after t i drives the motion of the bound H 2 + electron (transparent sky-blue blob). When the field becomes too weak to drive it over the barrier between well separated H + nuclei, it localizes at one of them to form an H atom at the time t frag . In this paper, for a given molecular orientation, we show that the phase of the laser field at the ionization instant strongly affects the choice of the nuclear site at which the bound electron localizes. Its influence in directing a bound electron to a particular direction along the internuclear axis is reflected in phase- and energy-dependent anisotropies in the angular distribution of emitted protons. 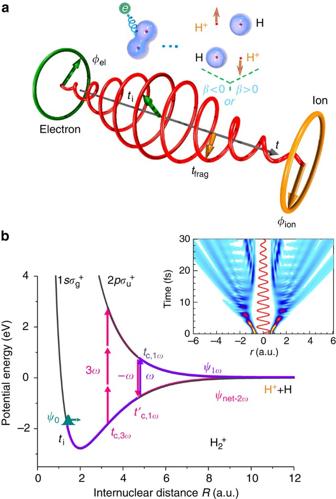Figure 1: Phase-dependent electron localization in molecular breakup. (a) The laser phase at ionization timetiis mapped to the electron emission angleϕelrecorded at one detector (green circle), and the alignment of the molecular axis is retrieved from the ion ejection angleϕionrecorded at the other (orange circle).ϕelis rotated by 90°with respect to the field- and tunnel-direction attidue to angular streaking. (b) Potential energy curves showing dissociation dynamics of the singly ionized H2+. Inset: Calculated time evolution of the probability of an H atom forming on the left or the right during H2+dissociation in laser field (red curve). Figure 1: Phase-dependent electron localization in molecular breakup. ( a ) The laser phase at ionization time t i is mapped to the electron emission angle ϕ el recorded at one detector (green circle), and the alignment of the molecular axis is retrieved from the ion ejection angle ϕ ion recorded at the other (orange circle). ϕ el is rotated by 90 ° with respect to the field- and tunnel-direction at t i due to angular streaking. ( b ) Potential energy curves showing dissociation dynamics of the singly ionized H 2 + . Inset: Calculated time evolution of the probability of an H atom forming on the left or the right during H 2 + dissociation in laser field (red curve). Full size image Angular streaking and coincident detection We use the rotating electric-field vector of the laser pulse as ultrafast clockwork and measure the asymptotic emission direction ϕ el of the tunnel-ionized electron. The value of ϕ el between 0 and 2 π provides the laser phase, relative to an arbitrary reference axis in the laboratory frame, at the ionization instant t i [10] , [11] , [12] , [13] , [14] , [15] . However, it is not ϕ el, but rather ϕ el mol , the phase of the laser field relative to the molecular axis at time t i , which determines the degree of anisotropy in bond breaking. The molecular-frame photoelectron angular distribution [16] has been widely used to probe the molecular geometry and dynamics. By assuming inversion symmetry, symmetric photoelectron angular distributions were expected and used to interpret the measured data [17] over the angular range of 0– π /2. In the present work, ϕ el mol is established by additionally determining the emission direction ϕ ion of the proton. ϕ ion reflects the alignment of the internuclear axis at time t i , as the time difference between the ionization and fragmentation, t frag − t i , is small relative to the rotational period of H 2 + and the momentum the proton acquires through dissociation dwarfs the momentum it gains from the laser field. The laboratory-frame angle difference ϕ el mol = ϕ el − ϕ ion between the electron and proton momentum vectors (or the electron emission angle in the molecular frame) is equal to the laser phase, in the molecular frame, at the time of ionization. In contrast to a ‘typical’ angular-streaking experiment in which time intervals are measured with attosecond resolution, ours is an energy- and angle-resolved measurement that determines the state of a system in the asymptotic limit of its time evolution. With respect to the measured asymmetric molecular-frame photoelectron angular distribution in a single symmetric synchrocyclotron pulse [18] , [19] , we observe asymmetric proton release in a single near-infrared multicycle circularly polarized pulse by tracking the electron localization in the molecular frame as a function of the laser phase at t i and the proton kinetic energy E k . Electron localization Electron localization in the breakup of hydrogen molecular ions has previously been observed [20] , [21] , [22] , [23] , [24] with symmetry-broken laser fields produced by CEP stabilizing a few-cycle pulse [20] , [21] , [22] or by composing a pulse of two different carrier frequencies [23] , [24] . The asymmetric fields drive and eventually localize the bound electron at one of the dissociating nuclei [25] . Alternatively, an attosecond pulse [26] , [27] , [28] is first used to launch a H 2 + vibrational wavepacket by single-photon ionization of H 2 . Next, a phase-locked near-infrared laser pulse drives the remaining electron back and forth between the nuclei until it localizes at one of them, the choice of localization site being dependent upon the delay between the excitation and the driving pulses. Such asymmetric electron localization was recently observed by measuring the released electron with a CEP-stabilized few-cycle pulse [29] or high-energy ultraviolet pulses in a pump-probe scheme [30] . The mechanism underlying electron localization in the present study can be understood as either the coherent superposition of the nuclear wavepackets of different inversion symmetry or, more intuitively, as the laser-driven motion of the remaining bound electron. In both pictures, the sign and magnitude of electron localization depends strongly on the laser phase ϕ i at the ionization instant and on the nuclear energy. Figure 1b shows a simplified potential energy diagram for H 2 + , comprising the two curves most relevant to the present study. A vibrational nuclear wavepacket on the 1 sσ g + curve is created by the early part of the laser pulse at time t i . The wavepacket is coupled forth-and-back between the 2 pσ u + and 1 sσ g + states at later times ( t c ) when the energy gap between the potential curves matches the photon energy (or three times the photon energy), with the molecular ion eventually dissociating into H + +H. Because of the coherent superposition of 1 sσ g + and 2 pσ u + contributions [20] , [21] , [22] , [23] , [24] , [25] , [26] , [27] , [28] , [29] , [30] , the electron probability density localizes asymmetrically at the nuclei. This electron localization dynamics is governed by the laser phase at the instant of field ionization ( t i ) and by the coupling times t c,3 ω , t c,1 ω and t ′ c,1 ω , which depend on the chosen photon energy and on the shape of the potential energy curves involved. As the energy gap between the potential curves depends on the internuclear distance, tuning the laser frequency changes the phase and energy dependence of electron localization. Similarly, different dependencies are to be expected for other molecules over a range of laser frequencies determined by their electronic structure. The inset in Fig. 1b shows the calculated time evolution of the probability of an H atom forming on the left or the right during H 2 + dissociation for a linearly polarized pulse. The present measurement does not determine this time evolution, but rather the phase and energy dependence of its asymptotic form. However, for completeness we note that a connection does exists between the angular information derived through our experiment and expressed through ϕ el mol , the laser phase ϕ i as referenced to the internuclear axis at the time of ionization t i and time differences between instants of ionization t i and electron localization t frag . To illustrate this, we denote T p as the period for one complete laser cycle (2.6 fs in the present case) and τ p as the laser pulse width (35 fs here) and refer again to Fig. 1a . For an arbitrary difference in electron and ion-emission angles ϕ el mol = ϕ i , the measured coincidence signal comprises the sum of all events occurring at the discrete times t frag − t i =( n+ϕ i /2 π ) T p where n =0,1,2,3… n f and n f ≤| τ p / T p |. In other words, it is sampled at discrete times described by a comb function whose sampling period correspond to T p . Thus, when signals for ϕ el mol = ϕ i and ϕ el mol = ϕ i +π are compared (as achieved through the asymmetry function defined in the next section), we are in fact comparing average localization rates for times determined by two comb functions displaced from one another by T p /2. Increasing the value of ϕ i from 0 to 2 π not only serves to delay the two measurement combs by T p from the ionization instant t i but also probes dissociation processes instigated by different field projections along the intermolecular axis. A COld Target Recoil Ion Momentum Spectroscopy (COLTRIMS) [31] reaction microscope is employed to measure, in time coincidence, the proton and electron produced by our 35-fs (~13.3 cycle at 790 nm) circularly polarized laser pulse and determine their momenta (see Methods). 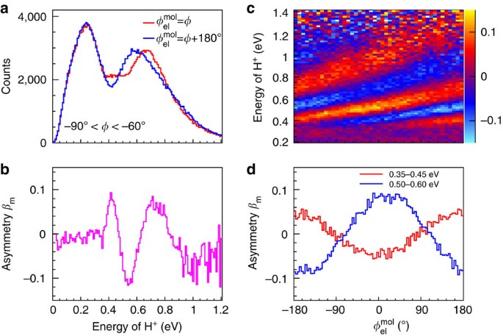Figure 2: Measured electron localization in dissociative single ionization of H2. (a) H+kinetic energy spectra following ionization by a 35-fs anticlockwise circularly polarized laser pulse (peak intensityI0=2.3 × 1014W cm−2). Curves shown forϕelmol=ϕandϕelmol=ϕ+180° where −90°<ϕ<−60°. (b) Molecular-frame asymmetry parameterβmversus H+kinetic energy for spectra plotted in (a). (c) Two-dimensional plot showingβmas a function of H+kinetic energy and the molecular-frame electron emission angleϕelmol. (d)βmversusϕelmolintegrated over H+kinetic energy intervals 0.35–0.45 eV (red curve) and 0.5–0.6 eV (blue curve). Asymmetric bond breaking Figure 2a shows two measured H + kinetic energy spectra for molecular-frame electron-emission angles ϕ el mol between −90° and −60° and between 90° and 120°. The 180° phase difference in ϕ el mol accounts for two dissociative single-ionization processes initialized with opposite laser field vectors. The two main proton energy peaks around 0.25 and 0.65 eV correspond to the one-photon (1 ω ) and net-two-photon (net-2 ω ) dissociation pathways ( Fig. 1b ), respectively. The kinetic energy spectrum shifts when ϕ el mol is changed by 180°. This is indicative of a kinetic-energy-dependent asymmetric dissociation or electron localization due to the interference between the 1 ω- and net-2 ω -dissociating wavepackets [20] , [21] , [22] , [23] , [24] , [25] , [26] , [27] , [28] , [29] , [30] , [32] . Figure 2: Measured electron localization in dissociative single ionization of H 2 . ( a ) H + kinetic energy spectra following ionization by a 35-fs anticlockwise circularly polarized laser pulse (peak intensity I 0 =2.3 × 10 14 W cm −2 ). Curves shown for ϕ el mol = ϕ and ϕ el mol = ϕ +180° where −90°< ϕ <−60°. ( b ) Molecular-frame asymmetry parameter β m versus H + kinetic energy for spectra plotted in ( a ). ( c ) Two-dimensional plot showing β m as a function of H + kinetic energy and the molecular-frame electron emission angle ϕ el mol . ( d ) β m versus ϕ el mol integrated over H + kinetic energy intervals 0.35–0.45 eV (red curve) and 0.5–0.6 eV (blue curve). Full size image To quantify the degree of localization, we define the molecular-frame asymmetry parameter as: where N ( ϕ el mol , E k ) is the H + yield at proton kinetic energy E k and electron angle ϕ el mol . The asymmetry parameter β m is positive for electron localization on one and negative for localization on the other nucleus, as illustrated in Fig. 1a . Figure 2b shows β m for the spectra in Fig. 2a . It oscillates as a function of E k with a modulation contrast of ~10%, about five times larger than reported in a recent pump-probe experiment [28] that employs an attosecond pulse train and a delayed infrared pulse. Figure 2c shows the dependence of β m on ϕ el mol and E k . The asymmetry changes over one period when ϕ el mol increases from −180° to 180° and is only significant in the energy range where contributions from the 1 ω and net-2 ω pathways overlap. This indicates that the coherent superposition of two states with different parity serves as the underlying mechanism for the observed electron localization. The phase dependence of the electron localization is further depicted in Fig. 2d , where different dependencies of β m on ϕ el mol are observed for two different proton kinetic energies. As discussed in the Supplementary Information , we confirmed the observed electron localization dynamics by switching the anticlockwise circularly polarized pulse to clockwise ( Supplementary Fig. S1 ), which can alternatively be probed in the laboratory frame ( Supplementary Fig. S2 ). Similar phase-dependent electron localization dynamics was also observed in D 2 ( Supplementary Fig. S3 ). To describe the experimental results, we employ two one-dimensional models that consider the component of the laser field along the direction of the molecular axis. In our semiclassical approach, we model the classical motion of the nuclei on the potential curves of H 2 + keeping track of the quantum phases. As illustrated in Fig. 1b , we start the nuclear motion on the 1 sσ g + potential surface at time t i and consider dissociation along two possible pathways: the 1 ω (violet curve) or the net-2 ω pathways (pink curve) (see Methods). We initialize the system with different kinetic energies at the equilibrium distance of H 2 (~1.4 a.u.) and add those trajectories that lead to the same final kinetic energy by taking into account their relative phases. 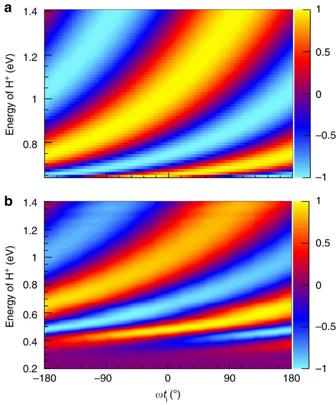Figure 3: Calculated electron localization in dissociative single ionization of H2. (a) Calculated asymmetry parameterβcas a function of the laser phaseωtiand the final kinetic energy of H+obtained from our classical model. (b) Same asabut for the asymmetry parameterβqobtained by numerically solving the one-dimensional time-dependent Schrödinger equation of the nuclear wavepacket. These results can be directly compared with the experimental results ofFig. 2c, as the molecular-frame electron emission angleϕelmolis a direct measure of the laser phaseωti. Figure 3a shows our semiclassically calculated asymmetry parameter β c as a function of the laser phase ωt i at the ionization instant and E k . Its predicted form is in good agreement with the experiment ( Fig. 2c ) for E k >0.6 eV. This confirms that our measured asymmetry is indeed due to interference between the 1 ω and net-2 ω dissociating wavepackets [20] , [21] , [22] , [23] , [24] , [25] , [26] , [27] , [28] , [29] , [30] , [32] . Figure 3: Calculated electron localization in dissociative single ionization of H 2 . ( a ) Calculated asymmetry parameter β c as a function of the laser phase ωt i and the final kinetic energy of H + obtained from our classical model. ( b ) Same as a but for the asymmetry parameter β q obtained by numerically solving the one-dimensional time-dependent Schrödinger equation of the nuclear wavepacket. These results can be directly compared with the experimental results of Fig. 2c , as the molecular-frame electron emission angle ϕ el mol is a direct measure of the laser phase ωt i . Full size image In our second two-state quantum mechanical model, we numerically solved the one-dimensional time-dependent Schrödinger equation for the vibrational nuclear wavepacket [33] (see Methods). The initial wavepacket in H 2 + is modelled assuming the molecular Ammosov-Delone-Krainov (ADK) tunnelling ionization rate for the depletion of the neutral H 2 in the laser field and is propagated along the two potential energy curves determined by the dipole coupling induced by the instantaneous laser field [34] . Figure 3b depicts the results from the quantum calculation, which again agree well in form with those of experiment ( Fig. 2c ) for the whole observed kinetic energy range. Our findings contrast the general belief that electron localization cannot be measured in symmetric laser fields, as represented by our single-carrier-frequency multicycle laser pulse. The data show that electron localization is not something that has to be artificially enforced by optical means [20] , [21] , [22] , [23] , [24] , [25] , [26] , [27] , [28] , but occurs naturally, even in pulses that are perfectly symmetric. Our technique, involving the coincidence detection of a streaked electron with a fragment ion, enables the phase and energy dependence of electron localization along a molecular bond to be explored in a transparent way. A key advantage of the present approach over others, where only one particle from a sequence of events is detected, is that phase resolution is not limited by the pulse width. Coincidence detection combined with angular streaking allows the determination of phase dependencies based on differences in momenta, which even for long pulses can be measured to high precision, providing a powerful tool for ultrafast science. Experimental technique We performed experiments with fs laser pulses (35-fs, 790 nm, 8 kHz) produced from a multipass amplifier Ti:sapphire laser system (KMLabs Dragon). The laser pulses were sent into a standard COld Target Recoil Ion Momentum Spectroscopy (COLTRIMS) setup [31] and focused by a concave reflection mirror with a focal length of 7.5 cm onto a supersonic gas jet. The jet is a mixture of H 2 and D 2 with a ratio of 1:1, so that both targets can be probed under identical conditions. The ions and electrons created by the laser were accelerated by a static electric field (~14.7 V cm −1 ) and detected by two-time and position-sensitive microchannel plate detectors [35] at opposite sides of the spectrometer. A weak homogeneous magnetic field (~9.2 Gauss) is used to enable the detection of the electron within a 4 π solid angle. The three-dimensional momentum vectors of the correlated ions and electrons are retrieved from the measured time-of-flight and position information during the offline analysis. We changed the polarization of the laser pulse from linear to circular by using a quarter waveplate with its fast axis orientated at 45° with respect to the input linear polarization. The handedness of the circular polarization can be switched from anticlockwise to clockwise by rotating the fast axis of the quarter waveplate by 90°. For the dissociative single-ionization channel H 2 →H+H + + e considered here, our apparatus could not measure the neutral H fragment. Thus, momentum conservation could not be invoked to suppress background signal by testing that the combined fragment momenta sum to zero. Nevertheless, the employment of a diffuse target jet and high-vacuum conditions led to extremely low event rates (~0.14 electrons per laser shot for the dissociative single-ionization channel), with the consequence that false background counts were reduced to <7% of the total counts for this channel. This false background slightly reduces the contrast in our derived asymmetries. Semiclassical model We propagate the nuclear wavepacket as a classical particle with reduced mass μ =0.5 on the unperturbed adiabatic potential energy curves and of H 2 + . Its motion follows Newton’s law and is driven by the force F =−∂ U /∂ R (ref. 36 ). As illustrated in Fig. 1b , the classical nuclear motion in the molecular ion is initiated at the equilibrium distance of the neutral molecule ( R 0 ~1.4 a.u.) at time t i with an initial energy of E 0 =U g0 +E k0 given by the sum of the potential and kinetic energy, named as E 0,1 ω and E 0,net-2 ω for the 1 ω and net-2 ω pathways, respectively. An initial kinetic energy (stemming from the finite width of the original wavepacket in momentum space) is given to the particle that allows it to reach the one-photon or three-photon energy gap where it is laser-coupled to the repulsive state. As illustrated in Fig. 1b , the two possible dissociation pathways are: the 1 ω pathway (violet curve; propagation on the 1 sσ g + , followed by coupling to the 2 pσ u + curve at time t c,1 ω by absorption of one laser photon, followed by dissociation along the 2 pσ u + curve) and the net-2 ω pathway (pink curve; propagation on the 1 sσ g + , followed by coupling to the 2 pσ u + curve at time t c,3 ω by absorption of three photons, followed by propagation on the 2 pσ u + curve and coupling back to the 1 sσ g + curve by emitting one photon at time t ′ c,1 ω , followed by dissociation along the 1 sσ g + curve). The accumulated phases of the wavepacket during the dissociation from R 0 to R inf from t i to t inf for these paths can be approximated as (in atomic units): where ϕ gu = π is the phase change due to coupling of the gerade state to the ungerade state and p ( R ) is the classical momentum associated with the wavepacket. The second term in the expression for ϕ 1 ω ( ϕ net−2 ω ) originates from the phase evolution of the laser pulse and is due to the absorption of one (three) photon. The fifth term in ϕ net-2 ω describes the emission of one photon. The probabilities for electron localization at the left or right nucleus are: By assuming | ψ 1 ω |=| ψ net−2 ω |, the asymmetry parameter within this semiclassical model is: Therefore, the asymmetrical electron localization due to interference between dissociating wavepackets on the 1 ω and net-2 ω pathways is governed by the phase difference between them. Figure 3a displays the semiclassically calculated asymmetry parameter β c as a function of the laser phase at ionization instant ωt i and the final kinetic energy E k , in good agreement with our measured asymmetry β m for E k >0.6 eV. The final kinetic energy from the 1 ω and net-2 ω pathways are E k,1 ω = E 0,1 ω + ω and E k,net-2 ω = E 0,net-2 ω +2 ω , respectively. Interference between the dissociated wavepackets requires equal final kinetic energy, corresponding to initial wavepacket energies for the two paths that differ by ω , that is, E 0,1 ω = E 0,net−2 ω + ω . This requirement and the applied initial kinetic energy give the lower limit of the final kinetic energy release in the classical calculation. To compare with the emission angles of the electron for circular polarization, the absolute phase of the laser is shifted by 90° in the simulation. This accounts for the 90° rotation of the electron angle with respect to initial tunnelling direction at the ionization instant due to the angular streaking of the circularly polarized pulse in the experiment. Quantum model The quantum dynamics of the nuclear wavepacket is modelled by solving the time-dependent Schrödinger equation within the subspace of the gerade (1 sσ g + ) and ungerade (2 pσ u + ) electronic states of H 2 + (ref. 33 ). Because mainly the laser polarization component parallel to the molecular axis influences the electron localization dynamics [20] , [21] , [22] , [23] , [24] , [25] , [26] , [27] , [28] , a simplified one-dimensional model is sufficient to reproduce the observed asymmetry in our experiment. The initial vibrational nuclear wavepacket in H 2 + is modelled based on molecular ADK rates for the depletion of the neutral hydrogen molecules as described in reference [34] . In brief, the ADK rate, which depends on the internuclear distance and instantaneous laser intensity, is integrated over time, divided by two and exponentiated to provide the R -dependent neutral-molecule-depletion factor d . The initial wavepacket in H 2 + is then obtained by multiplying the vibrational (and electronic) ground-state wavefunction of the neutral molecule with the factor (1- d ) followed by normalization of this product. The launch time defines the detected electron angle ϕ el and corresponds to the instantaneous ionization by the attosecond pulse in the two-colour pump-probe experiment [26] , [27] . After the wavepacket is launched, the remainder of the laser pulse is used to drive its motion. According to ADK rates, 94% of the ionization occurs in the seven most intense laser cycles around the pulse peak. The wavepackets launched during different laser cycles for the same laser phase (modulo 2 π ) are coherently added at the end of the propagation from the gerade ( ψ net-2 ω ) or ungerade ( ψ 1 ω ) potential curves, respectively. The probability for finding the electron localized at the left or right nucleus is calculated similar to the semiclassical model. Here, to determine the kinetic energy spectrum of the ion, we Fourier transform the dissociating parts of the nuclear wavepackets to obtain the momentum representations P ω ,l and P ω ,r , and calculate the asymmetry parameter as: Figure 3b depicts the simulated asymmetry parameter β q as a function of the laser phase at ionization time and the kinetic energy of the ion. The quantum mechanically calculated asymmetry parameter β q agrees well with the measured one, β m ( Fig. 2c ), except for the asymmetry contrast. The peak laser intensity in the simulation, adjusted to obtain the best agreement of the kinetic energy spectra, is I 0 =7.0 × 10 13 W cm −2 . It is lower compared with the peak intensity in experiment for the linear component along the molecular axis, which is 1.2 × 10 14 W cm −2 (we divided the peak intensity of the circularly polarized pulse by two to take into account the circular polarization). By using a lower value of peak intensity in the quantum simulation, we effectively average over the laser intensity profile in the experiment (focal-volume effect). How to cite this article: Wu, J. et al. Understanding the role of phase in chemical bond breaking with coincidence angular streaking. Nat. Commun. 4:2177 doi: 10.1038/ncomms3177 (2013).